The cholesterol transporter ABCG1 links cholesterol homeostasis and tumour immunity ATP-binding cassette transporter G1 (ABCG1) promotes cholesterol efflux from cells and regulates intracellular cholesterol homeostasis. Here we demonstrate a role of ABCG1 as a mediator of tumour immunity. Abcg1 −/− mice have dramatically suppressed subcutaneous MB49-bladder carcinoma and B16-melanoma growth and prolonged survival. We show that reduced tumour growth in Abcg1 −/− mice is myeloid cell intrinsic and is associated with a phenotypic shift of the macrophages from a tumour-promoting M2 to a tumour-fighting M1 within the tumour. Abcg1 −/− macrophages exhibit an intrinsic bias towards M1 polarization with increased NF-κB activation and direct cytotoxicity for tumour cells in vitro . Overall, our study demonstrates that the absence of ABCG1 inhibits tumour growth through modulation of macrophage function within the tumour, and illustrates a link between cholesterol homeostasis and cancer. In addition to the cancer cells and their surrounding stroma, the tumour microenvironment contains innate and adaptive immune cells that can recognize and destroy tumours [1] . However, the tumour not only manages to evade the immune system through various mechanisms, but also it contrives to benefit from infiltrating immune cells by modifying their functions to create a microenvironment favourable to tumour progression [2] . Macrophages are major players of tumour immunity. Monocyte-derived macrophages can polarize into either M1 (classically activated) or M2 (alternatively activated) macrophage subtypes in the presence of specific polarization factors, including cytokines, growth factors and bioactive lipids, when recruited into peripheral tissues [3] , [4] . In general, M1 macrophages are potent tumour-fighting cells, whereas M2 macrophages display protumoral functions. The tumour recruits blood monocytes and promotes their differentiation mostly into M2-like macrophages [5] . M2-like tumour-associated macrophages (TAMs) play a key role in tumour growth and progression by producing molecules to promote angiogenesis, as well as survival and metastasis of tumour cells [6] , [7] , [8] , [9] . Moreover, TAMs affect adaptive immune responses by recruiting T regulatory cells (Tregs), which in turn suppress antitumour effector cells such as NK cells and CD4 + /CD8 + T cells [10] . Several studies have reported a positive correlation between high TAM density and poor prognosis in human tumours, including bladder, breast and prostate [7] , [11] . Furthermore, it has been shown in different murine tumour models that either depletion of macrophages [12] , [13] , [14] , [15] , [16] or switching the phenotype of macrophages into tumour-fighting M1 macrophages [17] , [18] , [19] results in a significant reduction in tumour growth. ATP-binding cassette transporter G1 (ABCG1) is a member of the ABC transporter family that regulates cellular cholesterol homeostasis [20] . Cholesterol homeostasis is crucial for the survival and function of cells [21] . ABCG1 effluxes excess cholesterol from cells to high-density lipoprotein (HDL) particles for reverse cholesterol transport, which is the only path for elimination of cholesterol from the body [22] , [23] . ABCG1 is also important for the intracellular transport of cholesterol [24] , [25] . It is ubiquitously expressed in many cell types including myeloid cells, lymphocytes and endothelial cells [20] . ABCG1 is known to regulate several aspects of macrophage biology. Abcg1 −/− mice fed a Western-like diet display excessive lipid accumulation in macrophages [22] . Atherosclerosis studies demonstrated that ABCG1-deficient macrophages were more susceptible to apoptosis compared with wild-type (WT) macrophages under Western-like diet conditions in vivo [26] , [27] . Furthermore, Abcg1 −/− macrophages have been shown to display enhanced proinflammatory cytokine production at basal level [28] , [29] , in response to lipopolysaccharide (LPS) [30] and when loaded with cholesterol [31] . ABCG1 also plays a role in T-cell biology. We and others have reported that alterations in intracellular cholesterol homeostasis in the absence of ABCG1 increase proliferation of CD4 + T cells [32] , [33] and impairs development of invariant natural killer T cells in thymus [34] . Overall, changes in cholesterol homeostasis by the absence of ABCG1 modulate immune cell function; however, the role of ABCG1 in antitumour immune responses is unknown. In this study, we demonstrate that the in vivo deficiency of ABCG1 reduces tumour growth and increases the survival of mice. Reduced tumour growth in the absence of ABCG1 is mediated by myeloid cell intrinsic mechanisms and is associated with a shift of macrophages to a tumour-fighting M1 phenotype within the tumour, which results in the direct killing of tumour cells. ABCG1 deficiency prevents tumour growth in mice To determine if ABCG1 has an impact on tumour growth, MB49-bladder carcinoma or B16-F1 melanoma cells were first injected subcutaneously into 7–10-week-old Abcg1 −/− or control C57BL/6 (WT) mice fed a regular rodent chow diet (containing 0% cholesterol and 5% calories from fat; Fig. 1a ). Both groups of mice had comparable MB49 and B16-F1 tumour sizes when fed a chow diet ( Fig. 1b,c ). Because ABCG1 regulates cholesterol homeostasis in the cell, to make the impact of ABCG1 deficiency more prominent, 7–10-week-old Abcg1 −/− and WT mice were next fed a Western-like diet (containing 0.2% cholesterol and 42% calories from fat) beginning a week before MB49 or B16-F1 tumour inoculation. The Western-like diet used in our studies is very similar in cholesterol and fat content to the typical Western-like diet chosen by many people in developed countries, and now increasingly in developing countries. Abcg1 −/− mice fed a Western-like diet displayed dramatically reduced MB49 (fourfold at day 20) and B16-F1 (approximately threefold at day 20) tumour growth compared with control mice ( Fig. 1d,e ). By 6–8 months of age, Abcg1 −/− mice develop age-dependent phenotypes, such as pulmonary lipidosis and massive lipid deposition in macrophages [35] and these phenotypes are known to be accelerated by a Western-like diet [22] . Therefore, we also assessed the tumour growth in older (6–7 months old) Abcg1 −/− and WT mice fed a chow diet. Interestingly, we found that aged Abcg1 −/− mice when fed a chow diet had dramatically reduced MB49 tumour growth compared with aged-matched WT controls ( Fig. 1f ). 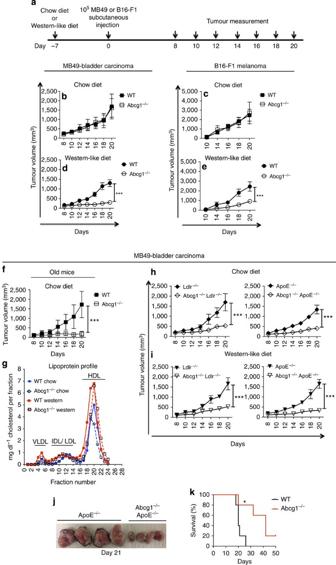Figure 1: ABCG1 deficiency reduces MB49 and B16 tumour growth. (a) Schematic diagram of the experimental design is shown. Graphs show (b) MB49 and (c) B16-F1 tumour growth in chow diet-fed and (d) MB49 and (e) B16-F1 tumour growth in Western-like diet-fed 7–10-week-oldAbcg1−/−(n=8) and C57BL/6 (WT) mice (n=8) and (f) MB49 tumour growth in chow diet-fed 6–7-month-oldAbcg1−/−(n=6) and WT (n=7) mice. (g) Blood plasma from five tumour-bearing mice for each group was pooled and the lipoprotein profile was analysed by fast protein liquid chromatography. Graph shows VLDL, IDL/LDL and HDL levels in all groups. (h–j) Graphs show MB49 tumour growth in (h) chow diet-fed and (i) Western-like diet-fedAbcg1−/−Ldlr−/−(n=6),Ldlr−/−(n=5);Abcg1−/−ApoE−/−(n=8) andApoE−/−(n=8) mice. (j) Picture shows harvested tumour masses from Western-like diet-fedAbcg1−/−ApoE−/−andApoE−/−mice at day 21. Data are representative of two to four independent experiments with similar results. (mean±s.e.m., ***P<0.001, two-way analysis of variance test). (k) Graph shows Kaplan–Meier survival curve of Western-like diet-fed tumour (MB49)-bearingAbcg1−/−(n=5) and WT mice (n=5). Data are representative of two independent experiments with similar results (mean±s.e.m., *P<0.05, log-rank test). IDL, intermediate-density lipoprotein; LDL, low-density lipoprotein; VLDL, very low-density lipoprotein. Figure 1: ABCG1 deficiency reduces MB49 and B16 tumour growth. ( a ) Schematic diagram of the experimental design is shown. Graphs show ( b ) MB49 and ( c ) B16-F1 tumour growth in chow diet-fed and ( d ) MB49 and ( e ) B16-F1 tumour growth in Western-like diet-fed 7–10-week-old Abcg1 −/− ( n =8) and C57BL/6 (WT) mice ( n =8) and ( f ) MB49 tumour growth in chow diet-fed 6–7-month-old Abcg1 −/− ( n =6) and WT ( n =7) mice. ( g ) Blood plasma from five tumour-bearing mice for each group was pooled and the lipoprotein profile was analysed by fast protein liquid chromatography. Graph shows VLDL, IDL/LDL and HDL levels in all groups. ( h – j ) Graphs show MB49 tumour growth in ( h ) chow diet-fed and ( i ) Western-like diet-fed Abcg1 −/− Ldlr −/− ( n =6), Ldlr −/− ( n =5); Abcg1 −/− ApoE −/− ( n =8) and ApoE −/− ( n =8) mice. ( j ) Picture shows harvested tumour masses from Western-like diet-fed Abcg1 −/− ApoE −/− and ApoE −/− mice at day 21. Data are representative of two to four independent experiments with similar results. (mean±s.e.m., *** P <0.001, two-way analysis of variance test). ( k ) Graph shows Kaplan–Meier survival curve of Western-like diet-fed tumour (MB49)-bearing Abcg1 −/− ( n =5) and WT mice ( n =5). Data are representative of two independent experiments with similar results (mean±s.e.m., * P <0.05, log-rank test). IDL, intermediate-density lipoprotein; LDL, low-density lipoprotein; VLDL, very low-density lipoprotein. Full size image To investigate how Western-like diet affects the cholesterol profiles of tumour-bearing Abcg1 −/− and WT mice, we performed fast protein liquid chromatography analysis of plasma lipoprotein cholesterol profiles of MB49 tumour-bearing (day 12) 7–10-week-old Abcg1 −/− and WT mice fed either chow or Western-like diets. In line with the published literature on Abcg1 −/− mice [24] , [36] , plasma lipoprotein cholesterol profiles of tumour-bearing Abcg1 −/− and WT mice were similar. In addition, Western-like diet feeding increased plasma lipoprotein cholesterol levels in both groups of mice ( Fig. 1g ). To further investigate the impact of ABCG1 deficiency on tumour progression, we crossed Abcg1 −/− mice with apoE-deficient ( ApoE −/− ) [37] , [38] and LDL-receptor-deficient mice ( Ldlr −/− ) [39] , [40] . The ApoE −/− and Ldlr −/− models are two hypercholesterolemic mouse models that are widely used to study atherosclerosis. Both genotypes have high plasma cholesterol levels when fed a chow diet and show profoundly increased plasma cholesterol levels when fed a Western-like diet [37] , [38] , [39] , [40] , [41] . We first compared the plasma lipoprotein cholesterol profiles of MB49 tumour-bearing (day 12) 7–10-week-old Abcg1 −/− ApoE −/− mice with ApoE −/− mice and Abcg1 −/− Ldlr −/− mice with Ldlr −/− mice, all fed a chow diet. We found that the loss of ABCG1 had no impact on plasma lipoprotein profiles in tumour-bearing hypercholesterolemic mice ( Supplementary Fig. 1 ). We next measured subcutaneous tumour growth in Abcg1 −/− mice crossed with these hypercholesterolemic mouse models. Interestingly, both 7–10-week-old Abcg1 −/− Ldlr −/− and Abcg1 −/− ApoE −/− chow-fed mice showed dramatically reduced MB49 tumour growth compared with chow-fed control Ldlr −/− and ApoE −/− mice, respectively ( Fig. 1h ). Both genotypes also displayed a profound reduction in tumour growth when fed a Western-like diet ( Fig. 1i,j ). Collectively, these data show that Western-like diet feeding or crossing with hypercholesterolemic mice is necessary to observe the changes in tumour growth in young Abcg1 −/− mice, while this tumour phenotype is evident in aged Abcg1 −/− mice fed a chow diet. To investigate the impact of ABCG1 deficiency on spontaneous tumour metastasis, we utilized luciferase-expressing B16-F10 cells (B16-F10-luc2). B16-F10-luc2 cells were injected subcutaneously into Western-like diet-fed Abcg1 −/− or WT mice. B16-F10-luc2 tumours grew aggressively and by day 28, the difference in tumour growth between Abcg1 −/− and WT mice was significant, but not very prominent ( Supplementary Fig. 2 ). This aspect of B16-F10-luc2 tumour growth allowed us to choose mice for study that had similar-sized tumours. Lungs from mice with similar, but average, tumour sizes in both groups were analysed for spontaneous metastases of B16-F10 melanoma by bioluminescence imaging ex vivo ( Supplementary Fig. 2 ). Subcutaneous B16 transplants have been shown to spontaneously metastasize to lung [42] , [43] . Abcg1 −/− mice had significantly diminished tumour metastasis compared with WT mice ( Supplementary Fig. 2 ). Subsequently, we examined the impact of ABCG1 deficiency on survival of tumour-bearing mice. MB49 tumour-bearing Abcg1 −/− mice showed prolonged survival compared with WT mice when fed a Western-like diet ( Fig. 1k ). Collectively, these data demonstrate that in vivo deficiency of ABCG1 impairs tumour growth and increases animal survival. Reduction in tumours in Abcg1 −/− mice is immune mediated To determine if the impact of ABCG1 deficiency on tumour growth is mediated by immune cells, we used a bone marrow chimera approach. We measured MB49 tumour growth in Western-like diet-fed irradiated CD45.1 + B6.SJL (WT) mice, which were reconstituted with CD45.2 + Abcg1 −/− or CD45.1 + B6.SJL bone marrow ( Fig. 2a ). WT mice reconstituted with Abcg1 −/− bone marrow had a significant reduction in tumour growth over time compared with WT mice reconstituted with WT bone marrow ( Fig. 2b ), demonstrating that the impact of ABCG1 deficiency on tumour growth is immune cell mediated. 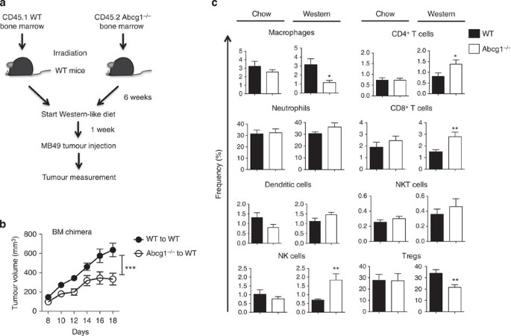Figure 2: Impact of ABCG1 deficiency on tumour growth is immune cell mediated. (a,b) Bone marrow chimeras were generated by reconstituting irradiated B6.SJL mice (n=16 total) with bone marrow cells from CD45.1+B6.SJL (WT) or CD45.2+Abcg1−/−donor mice. (a) Schematic diagram of the experimental design is shown. (b) Graph shows MB49 tumour growth in the chimeric mice. Data are representative of two independent experiments with similar results (***P<0.001, two-way analysis of variance test). (c) Tumour cells fromAbcg1−/−and C57BL/6 (WT) mice (n=5–7 per group) were analysed by flow cytometry 20 days after injection of MB49 cells. Bar graphs show the frequencies of macrophages, neutrophils, DCs, NK cells, CD4+T cells, CD8+T cells, NKT cells (% of live cells) and Tregs (% of CD4+T cells) in the tumour. (See methods andSupplementary Fig. 2for gating strategies). Data are pooled from two independent experiments with similar results (mean±s.e.m., *P<0.05, **P<0.01, two-tailed Student’st-test). Figure 2: Impact of ABCG1 deficiency on tumour growth is immune cell mediated. ( a , b ) Bone marrow chimeras were generated by reconstituting irradiated B6.SJL mice ( n =16 total) with bone marrow cells from CD45.1 + B6.SJL (WT) or CD45.2 + Abcg1 −/− donor mice. ( a ) Schematic diagram of the experimental design is shown. ( b ) Graph shows MB49 tumour growth in the chimeric mice. Data are representative of two independent experiments with similar results (*** P <0.001, two-way analysis of variance test). ( c ) Tumour cells from Abcg1 −/− and C57BL/6 (WT) mice ( n =5–7 per group) were analysed by flow cytometry 20 days after injection of MB49 cells. Bar graphs show the frequencies of macrophages, neutrophils, DCs, NK cells, CD4 + T cells, CD8 + T cells, NKT cells (% of live cells) and Tregs (% of CD4 + T cells) in the tumour. (See methods and Supplementary Fig. 2 for gating strategies). Data are pooled from two independent experiments with similar results (mean±s.e.m., * P <0.05, ** P <0.01, two-tailed Student’s t -test). Full size image The tumour microenvironment contains innate and adaptive immune cells, which display pro or antitumour functions. While NK cells, M1 macrophages, CD4 + Th1 cells and CD8 + T have been shown to act as tumour-fighting cells, M2 macrophages and Tregs in tumour are known to support tumour progression. Dendritic cells (DCs), neutrophils and NKT cells have been shown to exert both tumour-suppressive and -promoting effects [1] , [44] . Next we wanted to define the primary immune cell populations in the tumour microenvironment that are affected by the absence of ABCG1 under Western-like diet conditions. MB49 tumour cells were injected subcutaneously into either Western-like diet-fed or chow diet-fed Abcg1 −/− and WT mice and tumour-infiltrating immune cells were analysed by flow cytometry (For gating strategy, see Supplementary Fig. 3 ). We found that the frequencies of macrophages and Tregs significantly decreased, whereas the frequencies of NK cells, CD4 + T cells and CD8 + T cells significantly increased in the tumours of Western-like diet-fed Abcg1 −/− mice compared with WT mice ( Fig. 2c ). No significant differences were observed in the frequencies of tumour-infiltrating neutrophils, DCs or NKT cells in chow diet-fed or Western-like diet-fed Abcg1 −/− or WT mice ( Fig. 2c ). These results demonstrate that ABCG1 deficiency changes the balance between tumour-promoting and tumour-fighting immune cells within the tumour microenvironment. Tumour reduction in Abcg1 −/− mice is myeloid cell mediated To determine which cell type(s) were intrinsically affected by the absence of ABCG1 to impact tumour growth, we deleted ABCG1 selectively in either myeloid cells or T cells using Cre/loxP technology. We generated conditional knockout mice ( Abcg1 fl/fl ) in which loxP sites flank the Walker domain of exon 3 of Abcg1 and crossed them with either LysM-Cre or Lck-Cre mice for selective deletion of ABCG1 in myeloid cells and T cells, respectively [45] , [46] . We observed ~95% deletion of ABCG1 in macrophages from Abcg1 fl/fl -LysM-Cre + mice and 70% deletion of ABCG1 in T cells from Abcg1 fl/fl -Lck-Cre + mice ( Supplementary Fig. 4 ). We [32] and others [33] have previously reported that ABCG1 deficiency increases proliferation of CD4 + T cells. Therefore, it is possible that the impact of ABCG1 deficiency on tumour growth might be mediated directly through T-cell intrinsic mechanisms. To determine the impact of selective ABCG1 deletion in T cells on tumour growth, we injected MB49 tumour cells subcutaneously into Western-like diet-fed Abcg1 fl/fl -Lck-Cre + and control Abcg1 fl/fl -Lck-Cre − mice. The tumour growth in the Abcg1 fl/fl -Lck-Cre + mice was comparable to control ( Fig. 3a ), indicating that the inhibition of tumour growth in the absence of ABCG1 is not mediated directly through T cells. However, we found that the tumour growth in Abcg1 fl/fl -LysM-Cre + mice, which have selective ABCG1 deletion in myeloid cells, was dramatically reduced compared with control Abcg1 fl/fl -LysM-Cre − mice ( Fig. 3b ). These data indicate that the reduced tumour growth in the absence of ABCG1 is mediated directly through myeloid cell intrinsic mechanisms. 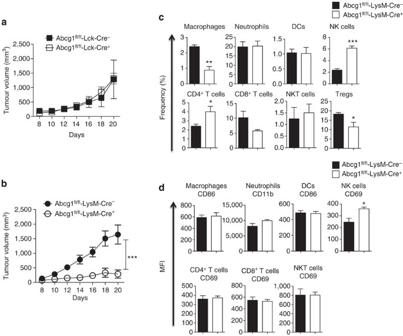Figure 3: Reduced tumour growth inAbcg1−/−mice is myeloid cell intrinsic. Graphs show MB49 tumour growth in Western-like diet-fed (a) Abcg1fl/fl-Lck-Cre+(n=7) and Abcg1fl/fl-Lck-Cre−(n=6) mice, (b) Abcg1fl/fl-LysM-Cre+(n=5) and Abcg1fl/fl-LysM-Cre−(n=7) mice. Data are representative of two independent experiments with similar results (***P<0.001, two-way analysis of variance test). Tumour cells from Western-like diet-fed Abcg1fl/fl-LysM-Cre+(n=5) and Abcg1fl/fl-LysM-Cre−mice (n=5) were analysed by flow cytometry 20 days after injection of MB49 cells. (c) Bar graphs show the frequencies of macrophages, neutrophils, DCs, NK cells, CD4+T cells, CD8+T cells, NKT cells (% of live cells) and Tregs (% of CD4+T cells) in tumour (See methods andSupplementary Fig. 2for gating strategies). (d) Bar graphs show the MFI of indicated activation markers on immune cells in the tumour. Data are representative of two independent experiments with similar results (mean±s.e.m., *P<0.05, **P<0.01, ***P<0.001, two-tailed Student’st-test). Figure 3: Reduced tumour growth in Abcg1 −/− mice is myeloid cell intrinsic. Graphs show MB49 tumour growth in Western-like diet-fed ( a ) Abcg1 fl/fl -Lck-Cre + ( n =7) and Abcg1 fl/fl -Lck-Cre − ( n =6) mice, ( b ) Abcg1 fl/fl -LysM-Cre + ( n =5) and Abcg1 fl/fl -LysM-Cre − ( n =7) mice. Data are representative of two independent experiments with similar results (*** P <0.001, two-way analysis of variance test). Tumour cells from Western-like diet-fed Abcg1 fl/fl -LysM-Cre + ( n =5) and Abcg1 fl/fl -LysM-Cre − mice ( n =5) were analysed by flow cytometry 20 days after injection of MB49 cells. ( c ) Bar graphs show the frequencies of macrophages, neutrophils, DCs, NK cells, CD4 + T cells, CD8 + T cells, NKT cells (% of live cells) and Tregs (% of CD4 + T cells) in tumour (See methods and Supplementary Fig. 2 for gating strategies). ( d ) Bar graphs show the MFI of indicated activation markers on immune cells in the tumour. Data are representative of two independent experiments with similar results (mean±s.e.m., * P <0.05, ** P <0.01, *** P <0.001, two-tailed Student’s t -test). Full size image Subsequently, we analysed the tumour-infiltrating immune cells in MB49 tumours from Western-like diet-fed Abcg1 fl/fl -LysM-Cre + and control mice by flow cytometry. In line with the changes in the frequencies of tumour-infiltrating immune cells in Western-like diet-fed Abcg1 −/− mice ( Fig. 2c ), the frequencies of tumour-infiltrating macrophages and Tregs in Abcg1 fl/fl -LysM-Cre + mice were significantly lower, whereas the frequencies of NK cells and CD4 + T cells were significantly higher compared with control ( Fig. 3c ). The frequencies of neutrophils, DCs, CD8 + cells and NKT cells in Abcg1 fl/fl -LysM-Cre + mice and control mice were comparable ( Fig. 3c ). We also analysed activation markers on tumour-infiltrating immune cells. We observed that the mean fluorescence intensity (MFI) of CD69 expression on NK cells was significantly higher in Abcg1 fl/fl -LysM-Cre + mice compared with control ( Fig. 3d ). The MFI of CD69 expression on CD4 + T cells, CD8 + T cells and NKT cells, the MFI of CD86 expression on macrophages and DCs and the MFI of CD11b expression on neutrophils were similar between both genotypes ( Fig. 3d ). LysM-Cre mice have been shown to display Cre-mediated deletion of loxP-flanked target genes in myeloid cells; mainly in macrophages and neutrophils and partially in DCs [46] . In both Western-like diet-fed Abcg 1 −/− mice and Abcg1 fl/fl -LysM-Cre + mice, the frequency of macrophages was decreased, whereas no significant differences were observed in the frequencies or the activation of tumour-infiltrating neutrophils and DCs ( Figs 2c and 3c,d ). Therefore, our data suggest that ABCG1 deficiency in macrophages likely promotes multiple antitumour immune responses. Impact of ABCG1 on apoptosis of tumour macrophages Next we investigated why ABCG1 deficiency caused a reduction in the frequency of macrophages in tumours. We first measured the frequency of monocytes in blood and in tumours from Abcg1 fl/fl -LysM-Cre + and Abcg1 fl/fl -LysM-Cre − mice fed a Western-like diet. The frequencies of monocytes in blood and tumours were similar in both groups ( Fig. 4a ), so changes in monocyte levels was not the cause. To determine if the reduction in the frequency of macrophages is due to an increase in macrophage cell death, we measured apoptosis of Abcg1 −/− and WT macrophages in the tumour by Annexin V staining and flow cytometry. We found that the percentage of apoptotic (Annexin V + live) macrophages in Western-like diet-fed Abcg1 −/− mice was significantly higher compared with WT mice ( Fig. 4b,c ). The percentage of apoptotic macrophages in chow diet-fed Abcg1 −/− and WT mice was comparable ( Fig. 4d,e ). These data show that macrophages in the tumour of Abcg1 −/− mice fed a Western-like diet display increased apoptosis. 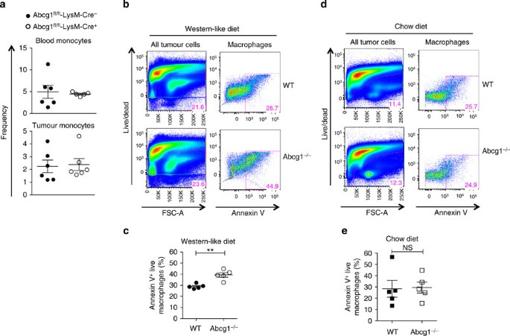Figure 4:Abcg1−/−macrophages in the tumour display enhanced apoptosis under Western-like diet conditions. (a) Blood and tumour cells from Western-like diet-fedAbcg1fl/fl-LysM-Cre+(n=6) andAbcg1fl/fl-LysM-Cre−(n=6) mice were analysed by flow cytometry 18 days after MB49 tumour injection. Dot plots show frequencies of monocytes (CD45+, NK1.1−, Ly6G−, CD11b+, CD115+; % of live cells) in blood (top) and tumour (bottom). (b–e) Tumour cells fromAbcg1−/−(n=5) and WT (n=5) mice were analysed for apoptosis by Annexin V staining and flow cytometry 12 days after injection of MB49 cells. (b,d) Representative pseudocolour plots show percentages of all tumour cells gated on live cells (left) and CD45+, NK1.1−, Ly6G−, CD11b+, F4/80highmacrophages, which are Annexin V+(right). Dot plots show the percentages of apoptotic (Annexin V+live) macrophages in tumours from (c) Western-like-diet-fed and (e) chow diet-fed mice. Data are representative of two independent experiments with similar results (mean±s.e.m., **P<0.01, two-tailed Student’st-test). Figure 4: Abcg1 −/− macrophages in the tumour display enhanced apoptosis under Western-like diet conditions. ( a ) Blood and tumour cells from Western-like diet-fed Abcg1 fl/fl -LysM-Cre + ( n =6) and Abcg1 fl/fl -LysM-Cre − ( n =6) mice were analysed by flow cytometry 18 days after MB49 tumour injection. Dot plots show frequencies of monocytes (CD45 + , NK1.1 − , Ly6G − , CD11b + , CD115 + ; % of live cells) in blood (top) and tumour (bottom). ( b–e ) Tumour cells from Abcg1 −/− ( n =5) and WT ( n =5) mice were analysed for apoptosis by Annexin V staining and flow cytometry 12 days after injection of MB49 cells. ( b , d ) Representative pseudocolour plots show percentages of all tumour cells gated on live cells (left) and CD45 + , NK1.1 − , Ly6G − , CD11b + , F4/80 high macrophages, which are Annexin V + (right). Dot plots show the percentages of apoptotic (Annexin V + live) macrophages in tumours from ( c ) Western-like-diet-fed and ( e ) chow diet-fed mice. Data are representative of two independent experiments with similar results (mean±s.e.m., ** P <0.01, two-tailed Student’s t -test). Full size image Abcg1 −/− macrophages shift towards an M1 phenotype Excess cholesterol is exported out of the cell by the cholesterol transporters ABCG1 and ABCA1 (refs 47 , 48 ). ABCG1 effluxes cholesterol to HDL particles [23] , while ABCA1 promotes cholesterol efflux to lipid-poor apolipoprotein AI (apoAI) [49] . We found that Abcg1 −/− macrophages expressed higher levels of Abca1 compared with WT macrophages in the tumour ( Supplementary Fig. 5 ). Subsequently, we investigated the phenotype of Abcg1 −/− macrophages in the tumour. We analysed the expression of CD11c, which is an M1-associated marker in tumour macrophages [50] . We found that in Western-like diet-fed Abcg1 −/− mice, the percentage of F4/80 high CD11c high (M1-like) macrophages was approximately five times higher than F4/80 high CD11c dim (M2-like) macrophages, whereas in WT mice the percentages of both groups were similar ( Fig. 5a,b ). Moreover, we found that in the chow diet-fed Abcg1 −/− mice, the percentage of F4/80 high CD11c high (M1-like) macrophages was only slightly (23%) higher than F4/80 high CD11c dim (M2-like) macrophages, whereas in WT mice the percentages of both groups were similar ( Supplementary Fig. 6 ). This shows that although Abcg1 −/− macrophages display a slight shift towards an M1 phenotype (based on CD11c high ) even under chow diet conditions, this phenotypic shift becomes much more prominent when the mice were fed with Western-like diet. To further analyse the polarization phenotype of tumour macrophages in Abcg1 −/− mice, we evaluated using quantitative real-time PCR the expression of M1 markers Tnfα and Nos2 and M2 markers Arg1 , Ccl22 and Mrc1 in macrophages sorted via flow cytometry from tumours from Western-like diet-fed Abcg1 −/− and WT mice. We found that the expression of Tnfα and Nos2 was significantly higher in tumour macrophages from Abcg1 −/− mice ( Fig. 5c ), whereas the expression of Arg1 , Ccl22 and Mrc1 was significantly lower in Abcg1 −/− macrophages compared with WT macrophages ( Fig. 5d ). These data point to a shift in the phenotype of macrophages in the tumours of Abcg1 −/− mice from tumour-promoting M2 macrophages to tumour-fighting M1 macrophages under Western-like diet conditions. 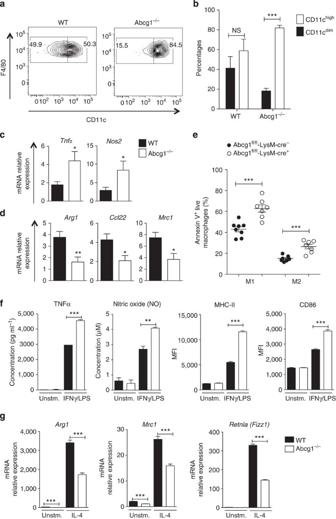Figure 5:Abcg1−/−macrophages shift towards an M1 phenotype in the tumour. (a,b) Tumour cells from Western-like diet-fedAbcg1−/−(n=6) and WT mice (n=6) mice were analysed by flow cytometry 20 days after injection of MB49 cells. (a) Representative contour plots and bar graphs show percentages of CD11chigh(M1-like) and CD11cdim(M2-like) macrophages (CD45+, NK1.1−, Ly6G−, CD11b+, F4/80high) in the tumour. (c,d) Macrophages were fluorescence-activated cell sorted from tumours from Western-like diet-fedAbcg1−/−and WT mice 20 days after inoculation of MB49 cells. Expression of (c) M1 markersTnfαandNos2and (d) M2 markersArg1, Ccl22, Mrc1were measured by quantitative real-time PCR (qPCR). (e) Tumour cells from Western-like diet-fedAbcg1fl/fl-LysM-Cre+(n=7) andAbcg1fl/fl-LysM-Cre−(n=8) mice were analysed for apoptosis by Annexin V staining and flow cytometry 12 days after injection of MB49 cells. Dot plot shows percentages of apoptotic (Annexin V+live) M1 (CD11chigh) and M2 (CD11cdim) macrophages in the tumour. Data are pooled from two independent experiments with similar results. (f,g) WT andAbcg1−/−BMDMs were polarized to an M1 phenotype by IFNγ/LPS stimulation or to an M2 phenotype by IL-4 stimulation,in vitro.Expression of (f) M1 markers and (g) M2 markers were analysed by enzyme-linked immunosorbent assay (ELISA) (TNFα), Griess reagent system (NO), flow cytometry (MHC II, CD86) or qPCR (Arg1, Mrc1, Retnla).Data are representative of two independent experiments with similar results (mean±s.e.m., *P<0.05, **P<0.01, ***P<0.001, two-tailed Student’st-test). Unstim., unstimulated. Figure 5: Abcg1 −/− macrophages shift towards an M1 phenotype in the tumour. ( a , b ) Tumour cells from Western-like diet-fed Abcg1 −/− ( n =6) and WT mice ( n =6) mice were analysed by flow cytometry 20 days after injection of MB49 cells. ( a ) Representative contour plots and bar graphs show percentages of CD11c high (M1-like) and CD11c dim (M2-like) macrophages (CD45 + , NK1.1 − , Ly6G − , CD11b + , F4/80 high ) in the tumour. ( c , d ) Macrophages were fluorescence-activated cell sorted from tumours from Western-like diet-fed Abcg1 −/− and WT mice 20 days after inoculation of MB49 cells. Expression of ( c ) M1 markers Tnfα and Nos2 and ( d ) M2 markers Arg1, Ccl22, Mrc1 were measured by quantitative real-time PCR (qPCR). ( e ) Tumour cells from Western-like diet-fed Abcg1 fl/fl -LysM-Cre + ( n =7) and Abcg1 fl/fl -LysM-Cre − ( n =8) mice were analysed for apoptosis by Annexin V staining and flow cytometry 12 days after injection of MB49 cells. Dot plot shows percentages of apoptotic (Annexin V + live) M1 (CD11c high ) and M2 (CD11c dim ) macrophages in the tumour. Data are pooled from two independent experiments with similar results. ( f , g ) WT and Abcg1 −/− BMDMs were polarized to an M1 phenotype by IFNγ/LPS stimulation or to an M2 phenotype by IL-4 stimulation, in vitro. Expression of ( f ) M1 markers and ( g ) M2 markers were analysed by enzyme-linked immunosorbent assay (ELISA) (TNFα), Griess reagent system (NO), flow cytometry (MHC II, CD86) or qPCR ( Arg1, Mrc1, Retnla). Data are representative of two independent experiments with similar results (mean±s.e.m., * P <0.05, ** P <0.01, *** P <0.001, two-tailed Student’s t -test). Unstim., unstimulated. Full size image We also analysed macrophages in the spleens and lungs of Western-like diet-fed MB49 tumour-bearing Abcg1 −/− and WT mice by flow cytometry at day 20. We found that Abcg1 −/− alveolar macrophages displayed enhanced MHC II expression compared with control, suggesting an M1 skewing. This result is consistent with the previous studies, which reported that Abcg1 −/− macrophages exhibited elevated proinflammatory activity in lung [28] , [29] . Although the level of MHC II expression in Abcg1 −/− spleen macrophages tended to be higher compared with control, it did not reach statistical significance ( Supplementary Fig. 7 ). Next we investigated why ABCG1-deficient macrophages shift towards an M1 phenotype in the tumour. Since we showed that Abcg1 −/− macrophages from Western-like diet-fed mice displayed increased apoptosis compared with WT macrophages ( Fig. 4b,c ), one possible explanation of this M1 shift could be that Abcg1 −/− M2 macrophages are more prone to apoptosis than Abcg1 −/− M1 macrophages. To test this, we measured apoptosis of both M1 and M2 macrophages in tumours from Western-like diet-fed Abcg1 fl/fl -LysM-Cre + and Abcg1 fl/fl -LysM-Cre − mice by Annexin V staining and flow cytometry. We found that M1 and M2 tumour macrophages from Abcg1 fl/fl -LysM-Cre + mice displayed similarly enhanced levels of apoptosis compared with control mice ( Fig. 5e ). Similar results for apoptosis were obtained also with staining for active Caspase-3 ( Supplementary Fig. 8 ). These data indicate that the shift towards M1 phenotype in the tumour on ABCG1 deficiency is not the result of M2 macrophages being more prone to apoptosis. Next we examined if Abcg1 −/− macrophages are intrinsically biased towards M1 polarization. To test this, we generated bone marrow-derived macrophages (BMDMs) from Abcg1 −/− and WT mice and polarized them to either an M1 phenotype by interferon-gamma (IFNγ)/LPS stimulation or to an M2 phenotype by interleukin-4 (IL-4) stimulation in vitro . First, we measured Abcg1 and Abca1 mRNA expression in polarized WT BMDMs. Both IFNγ/LPS and IL-4 stimulation significantly increased Abcg1 expression, but decreased Abca1 expression in WT macrophages ( Supplementary Fig. 9 ). Next we determined the expression of M1 and M2 markers in polarized Abcg1 −/− and WT BMDMs. We found that Abcg1 −/− macrophages had increased production of the M1 markers tumour-necrosis factor-α (TNFα; 50%) and nitric oxide (NO; 50%) after IFNγ/LPS stimulation compared with control ( Fig. 5f ). Moreover, Abcg1 −/− macrophages displayed enhanced expression of the M1 activation marker proteins MHC II (2.1-fold) and CD86 (~50%) when stimulated with the M1 inducers IFNγ/LPS ( Fig. 5f ). In contrast, Abcg1 −/− macrophages displayed decreased expression of the M2 markers Arg1 (twofold), Mrc1 (40%) and Retnla (Fizz1; 2.3-fold) after stimulation with the M2 inducer IL-4 ( Fig. 6g ). Arg1 (~20-fold) and Mrc1 (approximately twofold) expression levels were also significantly lower in non-polarized (unstimulated) Abcg1 −/− macrophages ( Fig. 5g ). These data indicate that Abcg1 −/− macrophages exhibit an intrinsic bias towards M1 polarization. Altogether these data show that the M1 shift of the Abcg1 −/− macrophages in the tumour is not due to increased apoptosis of M2 macrophages, but rather that Abcg1 −/− macrophages are biased toward M1 polarization. 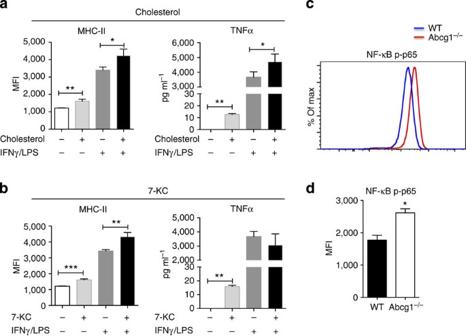Figure 6: Cholesterol and 7-KC stimulation increase expression of M1 markers in macrophages. (a,b) WT BMDMs were preincubated with cholesterol (20 μg ml−1) or 7-KC (5 μM) for 2 h. After that, the cells were stimulated with IFNγ (20 ng ml−1) and LPS (100 ng ml−1) or left unstimulated as described in the Methods. MHC II expression was analysed by flow cytometry and TNFα production was analysed by enzyme-linked immunosorbent assay. (c) Representative plot and (d) graph show levels of NF-κB p65 phosphorylation (Ser 529) inAbcg1−/−and WT BMDMs analysed by flow cytometry. Data are representative of two independent experiments with similar results. (mean±s.e.m., *P<0.05, **P<0.01, ***P<0.001, two-tailed Student’st-test). Figure 6: Cholesterol and 7-KC stimulation increase expression of M1 markers in macrophages. ( a , b ) WT BMDMs were preincubated with cholesterol (20 μg ml −1 ) or 7-KC (5 μM) for 2 h. After that, the cells were stimulated with IFNγ (20 ng ml −1 ) and LPS (100 ng ml −1 ) or left unstimulated as described in the Methods. MHC II expression was analysed by flow cytometry and TNFα production was analysed by enzyme-linked immunosorbent assay. ( c ) Representative plot and ( d ) graph show levels of NF-κB p65 phosphorylation (Ser 529) in Abcg1 −/− and WT BMDMs analysed by flow cytometry. Data are representative of two independent experiments with similar results. (mean±s.e.m., * P <0.05, ** P <0.01, *** P <0.001, two-tailed Student’s t -test). Full size image Abcg1 −/− macrophages accumulate cholesterol and cholesterol derivatives, such as 7-ketocholesterol (7-KC) [22] , [51] . To investigate if cholesterol and cholesterol derivatives have any impact on the M1 phenotype in macrophages, we incubated WT BMDMs with cholesterol and other sterols, including 7α-hydroxycholesterol (7α-OHC), 25-hydroxycholesterol (25-OHC), 27-hydroxycholesterol (27-OHC), desmosterol and 7-KC. After that, we either polarized BMDMs to an M1 phenotype by IFNγ/LPS stimulation or left them unstimulated. We found that incubation with cholesterol or 7-KC increased the levels of M1 markers, MHC II and TNFα in unstimulated macrophages. Incubation with cholesterol, but not 7-KC, also increased the levels of MHC II and TNFα after IFNγ/LPS stimulation ( Fig. 6a,b ). Incubation with 7α-OHC, 25-OHC, 27-OHC or desmosterol did not significantly alter the expression of M1 markers in either unstimulated or IFNγ/LPS- stimulated macrophages (data not shown). Thus, WT macrophages display an increase in the levels of M1 markers when incubated with cholesterol or 7-KC, suggesting that the M1-bias in Abcg1 −/− macrophages is likely due to the accumulation of these sterols. To better understand why Abcg1 −/− macrophages exhibit an intrinsic bias towards M1 polarization, we examined the activation of the transcription factor NF-κB, which is well established as playing a critical role in the induction of proinflammatory gene expression in macrophages [52] . Phosphorylation of p65 subunit of NF-κB helps stabilize NF-κB in the nucleus for gene transcription [53] and thereby is widely used as an indicator of NF-κB activation. We evaluated the levels of NF-κB p65 (Ser 529) phosphorylation in unstimulated Abcg1 −/− and WT BMDMs by flow cytometry. Abcg1 −/− macrophages showed an ~50% higher level of p65 phosphorylation compared with WT macrophages ( Fig. 6c,d ), indicating that the absence of ABCG1 results in an increased NF-κB activation in macrophages, which is a likely cause for the observed M1 phenotype bias. Abcg1 −/− macrophages show enhanced tumour cytotoxicity Next we investigated how the shift of macrophages towards an M1 phenotype in the absence of ABCG1 reduces tumour growth. M2-like TAMs support tumour growth through various mechanisms including promoting angiogenesis [6] , [7] , [8] , [9] Therefore, ABCG1 deficiency might decrease the ability of macrophages to promote tumour angiogenesis. To test this, we assessed the expression levels of endothelial cell markers in tumours from Abcg1 fl/fl -LysM-Cre + and Abcg1 fl/fl -LysM-Cre − mice by flow cytometry. We found comparable levels of CD45 − CD31 + CD34 + vascular endothelial cells in tumours from both mice groups ( Fig. 7a,b ), indicating that ABCG1-deficient macrophages are similar to WT macrophages in terms of promoting tumour angiogenesis, making this an unlikely mechanism. 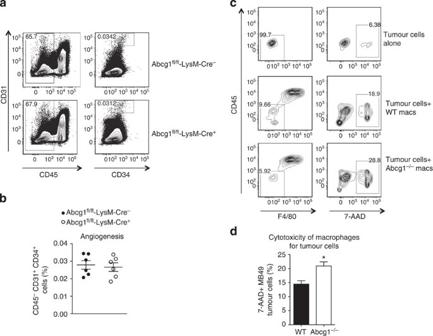Figure 7:Abcg1−/−macrophages display enhanced cytotoxicity for tumour cells. (a,b) Tumour cells from Western-like diet-fedAbcg1fl/fl-LysM-Cre+(n=6) andAbcg1fl/fl-LysM-Cre−(n=6) mice were analysed for angiogenesis markers by flow cytometry 18 days after injection of MB49 cells. (a) Representative contour plots and (b) dot plot show percentages of CD45−, CD31+and CD34+vascular endothelial cells in the tumour. (c,d) Cytotoxicity of macrophages for tumour cells was analysed by flow cytometry (See Methods). (c) Representative contour plots and (d) bar graph show percentages of CD45−, F4/80−, 7-AAD+MB49 tumour cells. Data are representative of two independent experiments with similar results (mean±s.e.m., *P<0.05, two-tailed Student’st-test). Figure 7: Abcg1 −/− macrophages display enhanced cytotoxicity for tumour cells. ( a , b ) Tumour cells from Western-like diet-fed Abcg1 fl/fl -LysM-Cre + ( n =6) and Abcg1 fl/fl -LysM-Cre − ( n =6) mice were analysed for angiogenesis markers by flow cytometry 18 days after injection of MB49 cells. ( a ) Representative contour plots and ( b ) dot plot show percentages of CD45 − , CD31 + and CD34 + vascular endothelial cells in the tumour. ( c , d ) Cytotoxicity of macrophages for tumour cells was analysed by flow cytometry (See Methods). ( c ) Representative contour plots and ( d ) bar graph show percentages of CD45 − , F4/80 − , 7-AAD + MB49 tumour cells. Data are representative of two independent experiments with similar results (mean±s.e.m., * P <0.05, two-tailed Student’s t -test). Full size image Unlike M2-like TAMs, M1 macrophages can be cytotoxic to tumour cells and, in this way, can prevent tumour growth [54] . To investigate if the impact of ABCG1 deficiency on tumour growth can be through increased ability of macrophages to kill tumour cells directly, we performed an in vitro cytotoxicity assay. In brief, we polarized bone marrow-derived Abcg1 −/− and WT macrophages to M1 phenotype by IFNγ/LPS stimulation and co-cultured these M1 macrophages with MB49 tumour cells. We assessed the viability of tumour cells by flow cytometry. We found that the frequency of dead tumour cells (CD45 − F4/80 − 7-AAD + ) was 40% higher when they were co-cultured with Abcg1 −/− macrophages, compared with WT macrophages ( Fig. 7c,d ). This indicates that Abcg1 −/− macrophages display enhanced cytotoxicity for tumour cells, making this a likely explanation for the reduced tumour growth observed in vivo . In this study, we identify a novel role for the cholesterol transporter ABCG1 as a modulator of tumour immunity. The absence of ABCG1 inhibits tumour growth through the modulation of macrophage survival and phenotype within the tumour. Collectively, our data demonstrate an important new concept that cholesterol homeostasis in immune cells can determine the outcome of tumour growth in vivo . LysM-Cre mice have been shown to display Cre-mediated deletion of loxP-flanked target genes in myeloid cells, mainly in macrophages and neutrophils and partially in DCs [46] . In tumours from Western-like diet-fed Abcg 1 −/− mice and Abcg1 fl/fl -LysM-Cre + mice, the frequency of macrophages was reduced, while the frequencies and the activation of neutrophils and DCs were similar compared with control ( Figs 2c and 3c,d ). Moreover, we showed that ABCG1-deficient macrophages exhibit an intrinsic bias toward tumour-fighting M1 polarization and display enhanced ability to kill tumour cells directly ( Fig. 7c,d ). Therefore, we conclude that the reduced tumour growth in the absence of ABCG1 is mediated through macrophage-intrinsic mechanisms. Increased apoptosis of Abcg1 −/− macrophages was also reported in atherosclerosis studies in mice, in which increased numbers of apoptotic macrophages were found within atherosclerotic lesions of Western-like diet-fed Abcg1 −/− ApoE −/− mice and Ldlr −/− mice transplanted with Abcg1 −/− bone marrow [26] , [27] . In addition, Abcg1 −/− macrophages have been shown to undergo apoptosis after a challenge with oxLDL [26] , [51] in vitro . Increased apoptosis of ABCG1-deficient macrophages is a result of the accumulation of specific toxic oxysterols, including 7-KC, which are known to induce apoptosis [27] , [51] . 7-KC and related oxysterols have been shown to be selectively exported out of the cell by ABCG1, but not by ABCA1 (ref. 51 ). Furthermore, the observed shift of Abcg1 −/− macrophages in the tumour towards a proinflammatory M1 phenotype ( Fig. 5a–d ) is in concordance with a previous study in atherosclerosis, which reported that macrophages from Abcg1 −/− mice fed a Western-like/high-cholesterol diet exhibited elevated proinflammatory activity [31] . Macrophages are known to accumulate cholesterol in the absence of ABCG1 (ref. 22 ). Our data demonstrate that macrophages display an increase in the levels of M1 markers when incubated with cholesterol or 7-KC ( Fig. 6a,b ), suggesting that the M1-bias in Abcg1 −/− macrophages is likely due to the excess sterol accumulation. In addition, similar to a previous report, which showed enhanced content of nuclear NF-κB p65 in Abcg1 −/− peritoneal macrophages after LPS stimulation [30] , we observed elevated NF-κB p65 phosphorylation in Abcg1 −/− BMDMs ( Fig. 6c,d ). A previous study by Li et al. [55] reported that free cholesterol accumulation in macrophages induced the production of proinflammatory cytokines through the activation of IκB kinase/NF-κB pathway. Therefore, based on our data, we surmise that an increased cholesterol accumulation in macrophages in the absence of ABCG1 causes NF-κB activation, which polarizes these macrophages to a proinflammatory/tumour-fighting M1 phenotype. M1 macrophages produce TNFα and NO, which can mediate cytolysis of tumour cells [54] . Thus, the enhanced production of TNFα and NO in Abcg1 −/− M1 macrophages that we reported here ( Fig. 5c,f ) is likely the cause of the observed increase in direct cytotoxicity of Abcg1 −/− macrophages for tumour cells ( Fig. 7c,d ). In most tumour models, the majority of the macrophages in tumours display a tumour-promoting M2 phenotype [5] . Our study shows that ABCG1 deficiency not only reduces the number of macrophages within the tumour, but also causes a shift of the remaining macrophages to a tumour-fighting M1 phenotype. Therefore, ABCG1 may constitute a therapeutic target for cancer. TAMs can promote tumour growth by different mechanisms. Production of CCL22 by immunosuppressive TAMs has been shown to recruit tumour-promoting Tregs to the tumour site [10] . Thus, our observation of reduced Treg frequency in the tumour in the absence of ABCG1 could be explained by a reduction in the frequency of TAMs ( Figs 2c and 3c ) and a phenotypic shift of the remaining TAMs to M1 macrophages, which are not potent CCL22 producers ( Fig. 5c,d ). Tregs suppress the expansion of antitumour effector cells including NK cells and CD4 + T cells [10] . Therefore, our observation of an increase in the frequency of NK cells and CD4 + T cells in the absence of ABCG1 could be explained by a decrease in the frequency of Tregs in the tumour ( Figs 2c and 3c ). Our data support the notion that M1 phenotypic shift of Abcg1 −/− macrophages with reduced CCL22 production results in reduced Treg recruitment, which in turn increases tumour infiltration by NK cells and CD4 + T cells. Since these cells are well-established tumour-fighting cells [1] , an increase in their frequency would have an impact on tumour growth. Collectively, our data support the concept that the absence of ABCG1 in macrophages drives changes in macrophage-intrinsic cytokine production and as such, could increase NK cell and CD4 + T-cell infiltration into the tumour to further prevent tumour growth. Our study suggests that intrinsic loss of ABCG1 in macrophages is of critical importance for the mechanisms behind the effects on tumour growth. Our data support the notion that accumulation of cholesterol in macrophages in the absence of ABCG1 impacts their survival and phenotype, thus changing their function in the tumour. Since Abcg1 −/− macrophages cannot efflux cholesterol properly, more cholesterol accumulates in Abcg1 −/− macrophages compared with WT macrophages, which has been well documented [22] . In young Abcg1 −/− mice, macrophage cholesterol accumulation is accelerated by Western-like diet feeding or by crossing the mice onto a hypercholesterolemic mouse model background. However, our finding that aged Abcg1 −/− mice display reduced tumour growth when fed a chow diet supports the notion that macrophages in older Abcg1 −/− mice accumulate more cholesterol over time [44] . Thus, in the aged Abcg1 −/− mice, the tumour phenotype becomes evident even on a chow diet. Enhanced expression of ABCG1 but reduced expression of ABCA1 after LPS/IFNγ or IL-4 stimulation in WT macrophages ( Supplementary Fig. 9 ) point to an importance of ABCG1 in macrophage activation. Increased expression of ABCA1 in Abcg1 −/− TAMs is not surprising ( Supplementary Fig. 5 ), since we [32] , [34] and others [36] , [56] have previously shown that genetic deletion of one cholesterol transporter, either ABCG1 or ABCA1, is compensated for by an upregulation of the other transporter. Nevertheless, neither ABCG1 nor ABCA1 can fully compensate for the loss of the other [20] . However, we cannot rule out the possibility that changes in ABCA1 expression contributed to our observed findings of reduced tumour growth in Abcg1 −/− mice. Future studies using ABCA1-deficient mice will be useful to delineate the roles of these two transporters in tumour immunity. From many perspectives, atherosclerosis and cancer are fundamentally different. However, the immune system plays a major role in the progression of both diseases. Human population and animal studies clearly demonstrate that HDL protects against atherosclerosis [57] . Interestingly, meta-analysis of lipid-altering therapies has indicated an inverse relationship between plasma HDL levels and incidence of cancer [58] . In concordance with this report, a recent study has shown that apoAI, the major protein component of HDL, suppresses tumour growth and metastasis in mice via the modulation of immune responses [59] . Collectively, these studies suggest that HDL has a role both in atherosclerosis and cancer. ABCG1 deficiency in immune cells has been shown to protect mice from atherosclerosis development [26] , [36] . By demonstrating that myeloid cell-specific ABCG1 deletion suppresses tumour growth, our present study suggests that ABCG1 might link immunity in atherosclerosis and cancer. In sum, our study identifies ABCG1 as a novel mediator of antitumour immune responses. It defines an important role for cholesterol transporters in tumour immunity and provides a link between lipid homeostasis and cancer. Understanding how ABCG1 and cholesterol metabolism in immune cells impacts antitumour immune responses could lead to development of entirely new therapeutic approaches for cancer immunotherapy. Mice C57BL/6J mice (000664), Ldlr −/− mice (002207) and ApoE −/− mice (002052) were purchased from The Jackson Laboratory (Bar Harbor, ME). Abcg1 −/− /lacZ knock-in mice were purchased from Deltagen (San Mateo, CA) and are congenic to a C57BL/6J background (backcrossed 14 generations). B6.SJL-Ptprca/BoyAiTac mice (CD45.1 congenic, 004007) were purchased from Taconic Farms (Germantown, NY). Abcg1 −/− mice were crossed with Ldlr −/− and ApoE −/− mice to obtain Abcg1 −/− Ldlr −/− and Abcg1 −/− ApoE −/− mice, respectively. Conditional knockout Abcg1 fl/fl mice (C57BL/6J background) in which loxP sites flank the Walker domain of exon 3 of Abcg1 were generated for our laboratory using InGenious Targeting Laboratory (New York). An ~10.3-kb region used to construct the targeting vector was first subcloned from a positively identified BAC clone using homologous recombination. The region was designed such that the short homology arm extends 2.2 kb 5′ to lox P/FRT-flanked Neo cassette. The long homology arm ends on the 3′ side of lox P/FRT-flanked Neo cassette and is ~8.1-kb long. The single lox P site is inserted upstream of exon 3, and the lox P/FRT-flanked Neo cassette is inserted downstream of exon 3. The target region is 1.5 kb including exon 3. The targeting vector is confirmed by restriction analysis after each modification step and by sequencing using primers designed to read from the selection cassette into the 3′ end of the long homology arm (N7) and the 5′ end of the short homology arm (N1), or from primers that anneal to the vector sequence, P6 and T7, and read into the 5′ and 3′ ends of the BAC sub clone. Abcg1 fl/fl mice were crossed with Lck-Cre mice (003802, The Jackson Laboratory) to obtain Abcg1 fl/fl -Lck-Cre + and control Abcg1 fl/fl -Lck-Cre − mice, and crossed with LysM-Cre mice (004781, The Jackson Laboratory) to obtain Abcg1 fl/fl -LysM-Cre + and Abcg1 fl/fl -LysM-Cre − mice. All the mice used in this study were female and 7–10 weeks old, except for the tumour growth experiment in the aged Abcg1 −/− and C57BL/6 (WT) mice, which were 6–7 months old. Mice were fed a standard rodent chow diet containing 0% cholesterol and 5% calories from fat (Pico lab, #5053) or Western-like diet containing 0.2% cholesterol and 42% calories from fat (Harlan Laboratories, #TD88137). The mice were housed in microisolator cages in a pathogen-free animal facility of the La Jolla Institute for Allergy and Immunology. The plasma lipid profile analyses were performed at day 12, because this is the very earliest time that significant differences were observed in tumour growth. Day 12 is also the time when differences in macrophage apoptosis were observed, which then later on leads to a more prominent difference in tumour growth. Tumour growth was measured until days 18–20 and that is the time when the frequency and phenotype of the immune cells within the tumour were analysed. All the experiments followed the guidelines of the La Jolla Institute for Allergy and Immunology Animal Care and Use Committee and approval for use of rodents was obtained from the La Jolla Institute for Allergy and Immunology according to criteria outlined in the Guide for the Care and Use of Laboratory Animals from the National Institutes of Health. Mice were euthanized by CO 2 inhalation. Cell lines and reagents MB49-bladder carcinoma and B16-F1 melanoma cells were derived from C57BL/6 mice and obtained from American Type Culture Collection. The B16-F10-luc2 cell line was established by Caliper Life Sciences by transduction of lentivirus containing luciferase 2 gene under the control of human ubiquitin C promoter. Tumour cells were cultured in R5 medium containing RPMI 1640, 5% heat-inactivated fetal bovine serum, 50 U ml −1 penicillin and 50 μg ml −1 streptomycin. Cells were injected into mice after reaching 60–80% confluency. Flow cytometry antibodies including anti-mouse APC-F4/80 (BM8; 1/100), FITC-Ly6G (RB6-8C5; 1/200), APC/Cy7 or AF700-CD45 (30-F11; 1/200), AF700-CD45.2 (104; 1/200), PerCP/Cy5.5-NK1.1 (PK136; 1/100), e-Fluor 450-CD4 (RM4-5; 1/200), FITC-TCRβ (H57-597; 1/400), PE-CD25 (PC61.5; 1/100), APC-Foxp3 (FJK-16s; 1/100), AF700-CD34 (RAM34; 1/200) and e-Fluor 450-MHC II (M5/114.15.2; 1/200), were purchased from eBioscience (San Diego, CA); PE-Cy7-CD11b (M1/70; 1/800), PE-CD11c (HL3; 1/300), FITC-CD45.1 (A20; 1/200), APC/Cy7-CD8α (53-6.7; 1/200), PE-Cy7-CD69 (H1.2F3; 1/400), PE-CD31 (MEC 13.3; 1/300) and PE-phospho-p65 (S529; K10-895.12.50; 1/10), were purchased from BD Biosciences (San Jose, California); PerCP/Cy5.5-CD19 (6D5; 1/100), PE-CD115 (AFS98; 1/100) and AF700-CD86 (GL-1; 1/200) were purchased from Biolegend (San Diego, CA). CD16/CD32 (2.4G2; 1/200) antibody was purchased from BD Biosciences. Ultrapure LPS ( Escherichia coli 0111:B4) was purchased from InvivoGen (San Diego, CA), murine rIFNγ and rIL-4 were purchased from R&D Systems (Minneapolis, MN), murine macrophage colony-stimulating factor (M-CSF) was purchased from PeproTech (Rocky Hill, NJ) and RPMI 1640 medium was purchased from Invitrogen (Carlsbad, CA). Fetal bovine serum, Collagenase IV, water-soluble cholesterol, 7α-OHC, 25-OHC, 27-OHC, desmosterol and 7-KC were purchased from Sigma-Aldrich (St Louis, MO). DNase I was purchased from Roche (Basel, Switzerland), PBS was purchased from Thermo Scientific (Rockford, IL) and Ficoll-Paque plus was purchased from GE Healthcare (Pittsburgh, PA). Measurement of tumour growth/metastasis and survival MB49 or B16-F1 cells (10 5 ) in 100 μl PBS were injected subcutaneously into the right flanks of female age-matched 7–10-week-old Abcg1 −/− , C57BL/6 (WT), Abcg1 −/− Ldlr −/− , Ldlr −/− , Abcg1 −/− ApoE −/− , ApoE −/− , Abcg1 fl/fl -Lck-Cre + , Abcg1 fl/fl -Lck-Cre − , Abcg1 fl/fl -LysM-Cre + and Abcg1 fl/fl -LysM-Cre − mice or 6–7-month-old Abcg1 −/− and WT mice. Mice were fed with either Western-like diet or chow diet beginning a week before injection of tumour cells. Tumour diameters were measured using a digital caliper and tumour volume was calculated using the formula V = D × d 2 /2, where V is the tumour volume, D is the largest measured tumour diameter and d is the smallest measured tumour diameter. For the survival experiments, the mice with tumour volume reaching 2,000 mm 3 were considered as dead and euthanized. To measure spontaneous lung metastasis, 10 5 luciferase-expressing B16-F10 cells (B16-F10-luc2) in 100 μl PBS were injected into female age-matched Abcg1 −/− and C57BL/6 mice subcutaneously. Mice were fed with Western-like diet beginning a week before injection of tumour cells. B16-F10-luc2 tumours grow more aggressively than B16-F1 tumours, which allowed us to choose mice for study that had similar-sized tumours. At 28 days after B16-F10-luc2 tumour inoculation, mice with similar, but average, tumour sizes in both groups were anaesthetized by inhalation of isoflurane (Butler Animal Health Supply) and 1 mg D -Luciferin (Caliper Life Sciences, Waltham, MA) in 100 μl PBS was delivered into each mouse retro-orbitally. Mice were euthanized 2 min after D -Luciferin injection, lungs were harvested and lung metastases were measured using an IVIS 200 Bioluminescence Imager (Caliper Life Sciences, Hopkinton, MA). Measurement of plasma lipoproteins Mice were fed with either chow diet or Western-like diet beginning a week before injection of tumour cells. Blood (in EDTA) was collected from chow diet-fed or Western-like diet-fed mice 12 days after MB49 tumour inoculation. Plasma lipoprotein profiles were obtained by fast protein liquid chromatography as described previously [60] , [61] . In brief, equal volumes of plasma from five mice per group were pooled and 200 μl of this pooled plasma was applied to a set of 2 Superose 6 (HR 10/30) columns linked in series. Lipoproteins were eluted by size exclusion into 0.5-ml fractions in EDTA/NaCl/NaN3 (1 mmol l −1 ; 0.154 mol l −1 ; 0.02%) at a flow rate of 0.5 ml min −1 . Cholesterol was measured in each fraction using an enzymatic cholesterol kit (Wako) according to the manufacturers’ instructions. Generation of bone marrow chimeras Recipient B6.SJL mice were irradiated in two doses of 500 rad each (for a total of 1,000 rad) 4 h apart. Bone marrow cells from both femurs and tibias of B6.SJL (CD45.1) and Abcg1 −/− (CD45.2) donor mice were collected under sterile conditions. Bones were centrifuged for the collection of marrow and the cells were washed and resuspended in PBS for injection. Bone marrow cells (10 7 ) from B6.SJL or Abcg1 −/− mice in 200 μl PBS were delivered retro-orbitally into each recipient mouse. Recipient mice were housed in a barrier facility under pathogen-free conditions and were provided autoclaved acidified water with antibiotics (trimethoprim-sulfamethoxazole) and were fed autoclaved food. The chimeric mice were fed with Western-like diet starting 6 weeks after bone marrow reconstitution. Flow cytometry Tumours were meshed through a 100-μm strainer (Fisher Scientific, Pittsburg, PA) and then filtered through a 40-μm strainer. Single-cell suspension was resuspended in 100 μl flow cytometry staining buffer (1% bovine serum albumin plus 0.1% sodium azide in PBS). Fcγ receptors were blocked with CD16/32-blocking antibody for 10 min and surface antigens on cells were stained for 30 min at 4 °C. LIVE/DEAD Fixable Dead Cell Stain (Invitrogen) was used for analysis of viability, and forward- and side-scatter parameters were used for exclusion of doublets from analysis. Antibody clones and dilutions used are listed above. For intracellular staining, cells were fixed and permeabilized with the Cytofix/Cytoperm Fixation/Permeabilization Solution Kit (BD Biosciences; for cytoplamis proteins) or Foxp3 Staining Buffer Set (eBioscience; for nuclear proteins) after the cell surface staining. Cells were stained with directly conjugated fluorescent of Foxp3 antibody for 30 min at 4 °C and with directly conjugated fluorescent of NF-κB phospho-p65 (Ser 529) antibody for 30 min at RT. Apoptosis of macrophages in tumour was measured by flow cytometry using a PE Annexin V Apoptosis Detection Kit 1 or a FITC active Caspase-3 Apoptosis Kit (BD Biosciences) according to the manufacturer’s instructions. Cell fluorescence was assessed using LSR-II (BD Biosciences) and data were analysed with FlowJo software (TreeStar, Ashland, OR). Macrophages (CD45 + , NK1.1 − , Ly6G − , CD11b + , F4/80 high ), neutrophils (CD45 + , NK1.1 − , Ly6G + , CD11b + ), myeloid DCs (CD45 + , NK1.1 − , Ly6G − , F4/80 − , CD11b + CD11c + ), monocytes (CD45 + , NK1.1 − , Ly6G − , CD11b + , CD115 + ), NK cells (CD45 + , TCRβ − , NK1.1 + ), CD4 + T cells (CD45 + , TCRβ + , NK1.1 − , CD4 + ), CD8 + T cells (CD45 + , TCRβ + , NK1.1 − , CD8 + ), NKT cells (CD45 + , TCRβ + , NK1.1 + ) and Tregs (CD45 + , TCRβ + , NK1.1 − , CD4 + ,CD25 + , Foxp3 + ) were identified with the appropriate gating. Cell sorting Tumours from WT and Abcg1 −/− mice at day 20 were enriched for CD11b + cells by positive selection with mouse CD11b + positive selection kit (Stem Cell Technologies, Vancouver, Canada) according to the manufacturer’s instructions, before cell sorting. Surface antigens on enriched CD11b + cells were then stained as described above, followed by macrophage (Ly6G − , NK1.1 − , CD11b + , F4/80 high ) sorting with a FACSAria cytometer (BD Biosciences). Peritoneal lavage from Abcg1 fl/fl -LysM-Cre + and Abcg1 fl/fl -LysM-Cre − mice 5 days post thioglycollate injection was sorted for macrophages (F4/80 high ) and splenocytes from Abcg1 fl/fl -Lck-Cre + and Abcg1 fl/fl -Lck-Cre − mice were sorted for T cells (CD3 + ) using FACSAria cytometer. Tumour angiogenesis Tumours were minced and digested with Collagenase IV (400 U ml −1 ) in the presence of DNase I (20 μg ml −1 ) in RPMI medium at 37 °C for 30 min. Cell suspension was filtered through a 40-μm strainer and resuspended in warm R5 medium and incubated at 37 °C for 30 min. The cells were stained with fluorophore-conjugated antibodies against CD45, CD31, CD34 and analysed by flow cytometry. Generation and M1/M2 polarization of BMDMs BMDMs were prepared as described previously [62] , [63] . In brief, bone marrow cells were cultured in standard tissue culture plates in the presence of 10 ng ml −1 M-CSF overnight. Non-adherent cells from this initial culture were then transferred to low-attachment six-well plates (Corning Life Sciences, Tewksbury MA) in 4 ml R5 medium containing 30% L929 conditioned medium and 10 ng ml −1 M-CSF per well for 7 days, adding more medium on days 3 and 6. After that, the cells were purified by centrifugation over Ficoll-Paque plus. Cells were verified to be 98% CD11b + , F4/80 + , MHC II low , CD80 low , CD86 low by flow cytometry. WT and Abcg1 −/− BMDMs were allowed to rest at 37 °C over night before stimulation. For M1 polarization, macrophages were either stimulated with IFNγ (20 ng ml −1 ) for 12 h followed by LPS (100 ng ml −1 ) stimulation for 4 h (for MHC II and CD86 analysis) or stimulated with IFNγ (20 ng ml −1 )+LPS (100 ng ml −1 ) overnight (for TNFα and NO analysis). For M2 polarization, macrophages were stimulated with IL-4 (20 ng ml −1 ) for 16 h. Stimulation of macrophages with cholesterol and -derivatives WT BMDMs were allowed to rest at 37 °C over night before stimulation. The next day, macrophages were preincubated with water-soluble cholesterol (20 μg ml −1 ), 7α-OHC (1 μM), 25-OHC (1 μM), 27-OHC (1 μM), desmosterol (5 μM) or 7-KC (5 μM) for 2 h. Next, macrophages were either left unstimulated or stimulated with IFNγ (20 ng ml −1 ) for 12 h followed by LPS (100 ng ml −1 ) stimulation for 4 h (for MHC II analysis) or stimulated with IFNγ (20 ng ml −1 )+LPS (100 ng ml −1 ) overnight (for TNFα analysis). Cytokine and NO measurements The supernatants were collected and TNFα was measured by ELISA (eBioscience) and NO (as nitrite) was measured by the Griess Reagent System (Promega, Madison, WI) according to the manufacturers’ instructions. In vitro tumour cytotoxicity assay WT and Abcg1 −/− BMDMs were plated in round well 96-well plates as 4 × 10 5 cells per well in 200 μl R5 and stimulated with IFNγ (20 ng ml −1 ) and LPS (100 ng ml −1 ) for 24 h. The cells were washed with R5 twice and co-cultured with 10 4 MB49 tumour cells (40:1 ratio of effector (macrophages): target cells (tumour cells) ). Twenty four hours later, the cells were washed with PBS and treated with Accutase cell detachment solution (BD Biosciences). Tumour cell viability was determined with 7-aminoactinomycin D (7-AAD) staining by flow cytometry. Tumour cytotoxicity was calculated as % of 7-AAD + tumour cells (CD45 − , F4/80 − ) co-cultured with macrophages (CD45 + , F4/80 + )—% 7-AAD + of tumour cells alone. Quantitative real-time PCR Total cellular RNA of macrophages was collected with an RNeasy Plus Micro Kit according to the manufacturer’s protocol (Qiagen, Valencia, CA). RNA purity and quantity was measured with a nanodrop spectrophotometer (Thermo Scientific). Approximately 500 ng RNA was used for synthesis of cDNA with an Iscript cDNA Synthesis Kit (Bio-Rad, Hercules, CA). Total cDNA was diluted 1:20 in H 2 O and a volume of 9 μl was used for each real-time condition with a MyIQ Single-Color Real-Time PCR Detection System (Bio-Rad) and TaqMan Gene Expression Mastermix and Arg1 (# Mm00475988_m1), Ccl22 (# Mm00436439_m1), Mrc1 (# Mm00485148_m1), Tnfα (# Mm00443258_m1), Rtnla (# Mm00445109_m1), Nos2 (# Mm00440502_m1), Abcg1 (# Mm01348250_m1) and Abca1 (# Mm01350760_m1) TaqMan primers (Applied Biosystems). Data were analysed and presented on the basis of the relative expression method [64] . The formula for this calculation is as follows: relative expression=2 −(SΔ Ct –CΔC t ) where Δ C t is the difference in the threshold cycle between the gene of interest and the housekeeping gene (18S), S is the Abcg1 −/− mouse and C is the WT mouse. Statistical analyses Data for all experiments were analysed with Prism software (GraphPad). Two-way analysis of variance test, long-rank test, unpaired Student’s t -test and Wilcoxon-matched-pairs signed rank test were used for comparison of experimental groups when appropriate. The data shown are the means±s.e.m. P values of less than 0.05 were considered statistically significant. How to cite this article: Sag, D. et al. The cholesterol transporter ABCG1 links cholesterol homeostasis and tumour immunity. Nat. Commun. 6:6354 doi: 10.1038/ncomms7354 (2015).